A wearable and highly sensitive pressure sensor with ultrathin gold nanowires Ultrathin gold nanowires are mechanically flexible yet robust, which are novel building blocks with potential applications in future wearable optoelectronic devices. Here we report an efficient, low-cost fabrication strategy to construct a highly sensitive, flexible pressure sensor by sandwiching ultrathin gold nanowire-impregnated tissue paper between two thin polydimethylsiloxane sheets. The entire device fabrication process is scalable, enabling facile large-area integration and patterning for mapping spatial pressure distribution. Our gold nanowires-based pressure sensors can be operated at a battery voltage of 1.5 V with low energy consumption (<30 μW), and are able to detect pressing forces as low as 13 Pa with fast response time (<17 ms), high sensitivity (>1.14 kPa −1 ) and high stability (>50,000 loading–unloading cycles). In addition, our sensor can resolve pressing, bending, torsional forces and acoustic vibrations. The superior sensing properties in conjunction with mechanical flexibility and robustness enabled real-time monitoring of blood pulses as well as detection of small vibration forces from music. Wearable and lightweight pressure sensing devices are of paramount importance for various future applications, such as electronic skin [1] , [2] , [3] , [4] , [5] , [6] , [7] , touch-on flexible displays [8] , [9] , soft robotics [10] , [11] and energy harvesting [12] , [13] , [14] . To date, pressure sensors are typically based on force-induced changes in capacitance [2] , [8] , [15] , [16] , piezoelectricity [17] , [18] , [19] , triboelectricity [7] , [13] and resistivity [20] , [21] . Recently, various nanomaterials, including nanowires [4] , [22] , [23] , carbon nanotubes [8] , [15] , [20] , polymer nanofibers [17] , [19] , [21] , [24] , metal nanoparticles [25] , [26] , [27] and graphene [28] have been used for the design of novel flexible pressure and strain sensors. The majority of these nanomaterials-based pressure sensors are based on capacitance or piezoelectricity except for a few recent reports [20] , [21] , where resistivity was used for designing strain gauge sensors. The advantage of resistive pressure sensors lies at simplicity in device fabrication as well as relatively low energy consumption in operation. Despite the promise, to date, only limited successful examples were reported on resistivity-based flexible pressure sensors [20] , [21] . The recently developed ultrathin gold nanowires (AuNWs) (~2 nm in width, with an aspect ratio of >10,000) [29] , [30] , [31] are mechanically flexible yet robust, enabling their uses in constructing novel superlattice nanomembranes [32] and flexible transparent electrodes [33] . Despite superior mechanical and electrical properties, ultrathin AuNWs have not yet been used in designing flexible sensors. Herein, we demonstrate that an AuNWs-impregnated tissue paper could be sandwiched between a blank PDMS sheet and a patterned PDMS sheet with interdigitated electrode arrays, leading to a superior wearable pressure sensor. Typically, a sensitivity of 1.14 kPa −1 could be achieved, which is comparable with the record in organic transistor pressure sensors reported recently [3] . Furthermore, our sensor could respond to pressure changes within 0.05 s at a frequency up to 5.5 Hz. We observed negligible loading–unloading signal changes over 50,000 cycles. Notably, the key sensing elements, AuNWs-impregnated tissue paper could be easily fabricated in large amount at low-cost using scalable wet chemistry processing steps. This enabled facile large-area fabrication and patterning for spatial pressure mapping. In addition, our AuNWs-based pressure sensors could be used to detect pressing, bending and torsional forces with high sensitivity, enabling their uses as wrist sensors and vibration sensors with low power consumption (<30 μW for an operating voltage of 1.5 V). These performances are comparable with the recently reported pressure sensing devices [3] , [5] , [6] , [7] , [13] , simultaneously offering advantages of low-cost and simplicity in device fabrication as well as versatility of detecting various force signals. 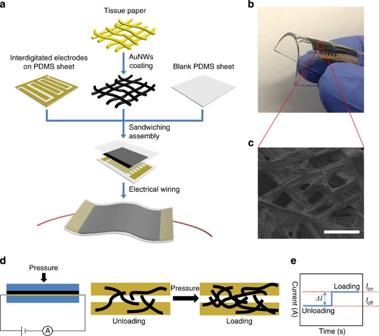Figure 1: Pressure sensor based on the AuNWs coated tissue paper. (a) Schematic illustration of the fabrication of a flexible sensor. (b) Photograph showing the bendability of the sensor. (c) Scanning electron microscopy image of the morphology of gold nanowires coated tissue fibres (scale bar, 100 μm). (d) Schematic illustration of the sensing mechanism. (e) Current changes in responses to loading and unloading (Ioff: unloading,Ion: loading). Device fabrication Figure 1a illustrates the fabrication process of our AuNWs-based pressure sensor. First, high-quality AuNWs were synthesized following the protocol reported recently [31] and concentrated to a stock solution of ~11 mg ml −1 . Note that AuNWs were ultrathin (only about 2 nm in width, comparable with the typical polymer chain width), yet tens of micrometres long, corresponding to an aspect ratio of >10,000. In addition, AuNWs were mechanically robust yet flexible, with curved structures without breaking [32] ( Supplementary Fig. 1 ). Figure 1: Pressure sensor based on the AuNWs coated tissue paper. ( a ) Schematic illustration of the fabrication of a flexible sensor. ( b ) Photograph showing the bendability of the sensor. ( c ) Scanning electron microscopy image of the morphology of gold nanowires coated tissue fibres (scale bar, 100 μm). ( d ) Schematic illustration of the sensing mechanism. ( e ) Current changes in responses to loading and unloading ( I off : unloading, I on : loading). Full size image Second, AuNWs were deposited into Kimberly-Clark tissue paper by simple dip-coating and drying. The dip-coating process was repeated for 10 times, giving a dark tissue paper with a sheet resistance of 2.5±0.4 MΩ sq −1 measured from 10 samples, and leading to an average off-resistance of 91.1±52 kΩ after their integration into pressure sensors ( Supplementary Fig. 2 ). Both optical microscopy and scanning electron microscopy demonstrated uniform deposition of AuNWs onto tissues papers ( Supplementary Fig. 3 ). Finally, the AuNWs-impregnated tissue paper was sandwiched between a blank 500 μm-thick PDMS sheet and a PDMS sheet patterned with interdigitated electrode arrays ( Supplementary Fig. 4 ). PDMS surfaces were treated by plasma before sandwiching, enabling their conformal contact and firm bonding with tissue paper ( Supplementary Fig. 5 ). Such fabricated devices are wearable and bendable due to the flexible nature of both tissue paper and AuNWs ( Fig. 1b,c ). The sensing mechanism is due to pressing force-dependent contact between AuNWs and interdigitated electrode arrays. Unlike a bulk rigid planar metal, soft tissue paper has porous and rough surfaces with hairy AuNWs. The number of AuNWs bridging finger electrode pairs depended on the external forces applied. On applying an external pressure, a small compressive deformation of tissue paper enabled more AuNWs in contact with finger electrodes, leading to more conductive pathways ( Fig. 1d ). This caused an increase in current when a fixed voltage of 1.5 V was applied ( Fig. 1e ). On unloading, both PDMS and tissue paper recovered to their original shapes, reducing the amount of AuNWs bridging the finger electrode pairs, therefore, leading to the decrease of the current. Cycling tests and sensitivity To measure the responses of our AuNWs-based sensors to both static and dynamic mechanical pressures, a home-made system containing a computer-controlled stepping motor and a force sensor were designed ( Fig. 2a ). Such a system can provide an external pressure of up to 50 kPa (static pressure) and 3 kPa (dynamic pressure) with electrical signals simultaneously recorded. Our AuNWs-based pressure sensor showed a steady response to static pressure up to 50 kPa and the resistance under each pressure was constant ( Supplementary Fig. 6 ). For dynamic force measurement, we performed multiple loading–unloading tests under various pressures at a frequency of 3 Hz. After ~10,000 cycles, the sensor performance showed little changes at various pressures ranging from 500–3,000 Pa ( Fig. 2b ). 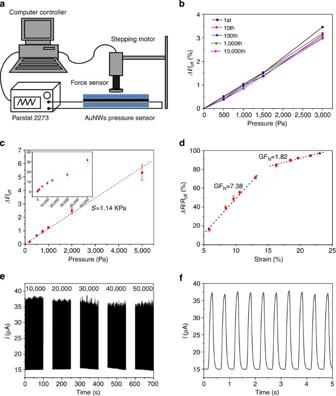Figure 2: Evaluation of sensing performances. (a) Schematic illustration of the experimental setup. (b) Sensitivity after repeated loading–unloading cycles at a frequency of 3 Hz. (c) Current response to various pressures. Dot line is a linear regression giving a sensitivity of ~1.14 kPa. (d) Electrical resistance changes under various strains. Gauge factor, GFNcould be derived by linear fitting. (e) The durability test under a pressure of 2,500 Pa at a frequency at 2 Hz. The current change curves were recorded after each 10,000 cycles and 200 cycles of data were presented in each recording. (f) Enlarged view of the part of theI–tcurve ineafter 10,000 loading–unloading cycles. Figure 2: Evaluation of sensing performances. ( a ) Schematic illustration of the experimental setup. ( b ) Sensitivity after repeated loading–unloading cycles at a frequency of 3 Hz. ( c ) Current response to various pressures. Dot line is a linear regression giving a sensitivity of ~1.14 kPa. ( d ) Electrical resistance changes under various strains. Gauge factor, GF N could be derived by linear fitting. ( e ) The durability test under a pressure of 2,500 Pa at a frequency at 2 Hz. The current change curves were recorded after each 10,000 cycles and 200 cycles of data were presented in each recording. ( f ) Enlarged view of the part of the I–t curve in e after 10,000 loading–unloading cycles. Full size image The sensitivity of our pressure sensor is defined as S =( ΔI / I off )/ ΔP , where ΔI is the relative change in current, I off is current of the sensor under no load and ΔP is the change in applied pressure. An approximately linear relationship between ΔI / I off and applied pressure P in the range of 0–5 kPa, leading to a sensitivity value S =1.14 kPa −1 . This value is only next to the record value in organic transistor pressure sensors [3] and higher than the typical sensitivity of 5 × 10 −3 –0.55 kPa −1 reported from other pressure sensors, which have a sensing area of 0.6 × 0.6 mm 2 –8 × 8 mm (refs 22 , 34 , 35 , 36 , 37 ). In addition, higher sensitivity could be achieved by further increasing the dip-coating cycles of AuNWs ( Supplementary Fig. 7 ) and reducing the PDMS thickness ( Supplementary Fig. 8 ). To assess the ability of our device to function as a strain gauge sensor, we measured the gauge factor (GF), which is usually defined as the ratio of relative change in electrical resistance ( ΔR / R off ) to the mechanical strain, ε . For our case, the forces were applied at normal directions, causing the thickness changes, ε N . Then, GF at the normal direction GF N =( ΔR / R off )/ ε N . As shown in Fig. 2d , the GF below the strain of 14% showed a higher linear slope of 7.38. In the high strain range (14–25%), the average GF dropped to 1.82. We further demonstrate high durability of our AuNWs pressure sensor under a pressure of 2,500 Pa at a frequency of 2 Hz ( Fig. 2e ). Note that the high signal-to-noise ratios were well maintained and the current amplitude exhibited negligible changes after 50,000 loading–unloading cycles. The high stability was also demonstrated in a bending test and the device sensitivity did not show evident changes after repeated bending for over 5,000 cycles at 30 mm radius of curvature ( Supplementary Fig. 9 ). Time-resolved responses To examine the response time of our sensors to external forces, the output current signals were compared with the dynamic pressure inputs at a frequency of 1–5.5 Hz ( Fig. 3 ). Note that the current waves were almost the same as the input pressure waves under a pressure of ~400 Pa at the lower frequency (1–2 Hz). Furthermore, the applied pressure was increased to 600 Pa at a frequency of 1, 3 and 5.5 Hz ( Fig. 3c ). The output electrical signals remained stable without evident change in amplitude up to 5.5 Hz. A negligible hysteresis was observed under a pressure of 600 Pa at 1 Hz ( Supplementary Fig. 10a,b ), which increased with the increasing frequency up to 0.05 s at 5.5 Hz. This hysteresis may be attributed to elastic deformation of tissue paper during loading–unloading process and the viscoelastic effects of the PDMS layers [21] . However, the bandwidth and the line shapes kept almost unchanged as the force frequency increased. Similar quick response time was also observed in the abrupt unloading process from 1,600 to 0 Pa ( Supplementary Fig. 10c ), where a response time of 17 ms was obtained. 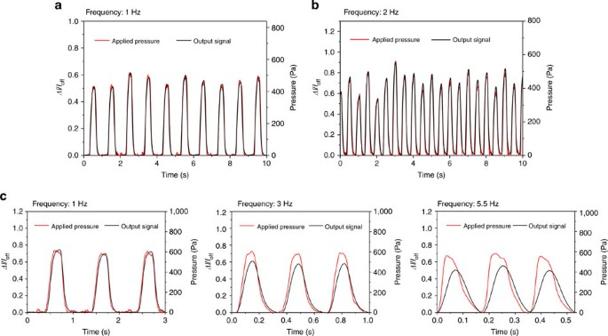Figure 3: Pressure-resolved and time-resolved responses. (a,b) Pressure-resolved measurements of the output signal as the function of applied pressure in the range of 400–550 Pa at the frequency of 1 Hz and 2 Hz, respectively. (c) Plots showing frequency responses at the dynamic pressure of 600 Pa: pressure input frequency of 1, 3 and 5.5 Hz. Figure 3: Pressure-resolved and time-resolved responses. ( a , b ) Pressure-resolved measurements of the output signal as the function of applied pressure in the range of 400–550 Pa at the frequency of 1 Hz and 2 Hz, respectively. ( c ) Plots showing frequency responses at the dynamic pressure of 600 Pa: pressure input frequency of 1, 3 and 5.5 Hz. Full size image Pressure-resolved responses To estimate the pressure range of our AuNWs-based sensors towards dynamic forces, a piezoelectric stepping positioner with minimum displacement of only 1 μm was applied to the sensors. As shown in Fig. 4a a pressure of 13 Pa could be detected, which is equivalent to the weight of a water droplet (~13 μl) on a surface of 10 mm 2 . At the higher pressure range, the noise-free, stable continuous responses could be observed up to 2,600 Pa ( Fig. 4b ). 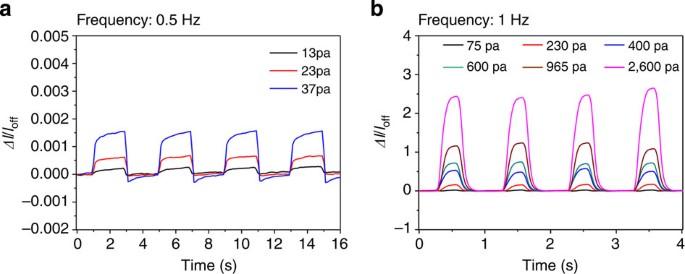Figure 4: Dynamic pressure response at low and high pressure range. (a) Plot of current response as a function of time (pressure input frequency: 0.5 Hz) for three applied pressures (13, 23 and 37 Pa). (b) Plot of current response of the sensor as a function of time (pressure input frequency: 1 Hz) for the applied pressures in the range of 75–2,600 Pa. Figure 4: Dynamic pressure response at low and high pressure range. ( a ) Plot of current response as a function of time (pressure input frequency: 0.5 Hz) for three applied pressures (13, 23 and 37 Pa). ( b ) Plot of current response of the sensor as a function of time (pressure input frequency: 1 Hz) for the applied pressures in the range of 75–2,600 Pa. Full size image Detection of other types of mechanical forces In addition to pressing forces, our pressure sensor can simultaneously be used to detect the bending and torsional forces. Remarkably, the response curves are characteristic for each kind of mechanical forces for the same device ( Fig. 5 and Supplementary Movie 1 ). High signal-to-noise ratios were observed in all the three types of force measurements, further demonstrating the high sensitivity of our AuNWs pressure sensor. The device also exhibited stable linear responses to various bending forces ( Supplementary Fig. 11 and Supplementary Table 1 ). 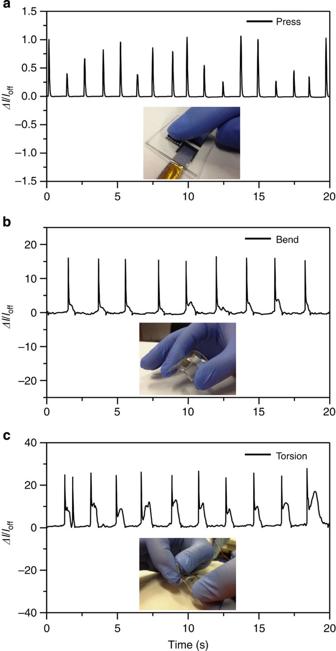Figure 5: Detection of other types of mechanical forces. (a–c) Plots showing the current responses to dynamic loading and unloading cycles: (a) pressing, (b) bending and (c) torsion. Figure 5: Detection of other types of mechanical forces. ( a – c ) Plots showing the current responses to dynamic loading and unloading cycles: ( a ) pressing, ( b ) bending and ( c ) torsion. Full size image Detection of wrist pulses Our AuNWs-based pressure sensors are wearable and could be used to monitor the blood pressure of a human radial artery in real-time ( Fig. 6a , Supplementary Fig. 12a and Supplementary Movie 2 ). The wrist pulses could be read out accurately under both normal condition (~66 beats per minute) and after physical exercise (~88 beats per minute) as shown in Fig. 6b . Note that the amplitude and frequency of pulses under two conditions were clearly different. Under normal condition, a typical radial artery pulse waveform was obtained with two clearly distinguishable peaks ( P 1 and P 3 ) and a late systolic augmentation shoulder ( P 2 ) ( Fig. 6c ). The line shape is known to be caused by constitution of the blood pressure from the left ventricle contracts and reflective wave from the lower body [38] . The radial augmentation index AI r = P 2 / P 1 is a characteristic value for arterial stiffness, which highly related to the age of people [38] . From a series of waveforms measured with our AuNWs-based pressure sensor, we estimated an average AI r of 0.7, agreeing quite well with the literature data [38] for a healthy 37-year-old male. After the physical exercise, the pulse wave shapes exhibited a change in which the late systolic augmentation ( P 2 ) disappeared. This could be due to a few reasons such as altered heart rate/ventricular ejection characteristics, large artery stiffness/PWV, or change in tone of muscular arteries influencing pressure wave reflection as described in the literature [39] . The above results demonstrate that the subtle differences in blood pulses could be identified with our AuNWs-based pressure sensors, indicating its potential to serve as a wearable diagnostic device to monitor human’s health in real-time under various conditions. 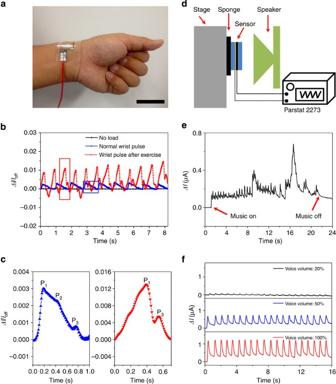Figure 6: Real-time andin-situartery wrist pulses and acoustic vibrations. (a) Photograph showing the skin-attachable sensor directly above the artery of the wrist (scale bar, 3 cm). (b,c) Measurement of the physical force of a heartbeat under normal (66 beats per minute) and exercise conditions (88 beats per minute). (d) Schematic illustration of the setup for acoustic vibration sensing. (e) The current responses to the acoustic vibrations from a piece of music. (f) The current responses to the acoustic vibrations from regularly clicking mouse. Note that three different voice volumes (20, 50, and 100%) were tested. Figure 6: Real-time and in-situ artery wrist pulses and acoustic vibrations. ( a ) Photograph showing the skin-attachable sensor directly above the artery of the wrist (scale bar, 3 cm). ( b , c ) Measurement of the physical force of a heartbeat under normal (66 beats per minute) and exercise conditions (88 beats per minute). ( d ) Schematic illustration of the setup for acoustic vibration sensing. ( e ) The current responses to the acoustic vibrations from a piece of music. ( f ) The current responses to the acoustic vibrations from regularly clicking mouse. Note that three different voice volumes (20, 50, and 100%) were tested. Full size image Detection of acoustic vibrations Our AuNWs-based could be also applied to detect acoustic vibrations. To prove such a capability, we attached our sensor to a sponge and positioned them close to a speaker with a fixed spacing from a few to tens of millimetres ( Fig. 6d ). Interestingly, the tiny vibrational forces from both music and repeated sounds could be accurately resolved ( Supplementary Fig. 12 and Supplementary Movies 3 and 4 ). Note that the reliable current signals accompanied to both amplitude and frequency of acoustic vibrations could be detected when the sensor was 30 mm away from the speaker. Even when the voice volume was decreased to 20%, the well-defined current waves could still be obtained ( Fig. 6f ). Large-scale integration and patterning Both synthesis of AuNWs and fabrication of AuNWs-impregnated tissue papers are essentially based on wet chemistry techniques and both are scalable, enabling facile large-scale integration and patterning. In a typical demonstration, we fabricated an AuNWs-impregnated tissue paper sheet of 5 × 5 cm 2 ( Fig. 7a ) and cut them into 25 pieces (4 × 5 mm 2 each) and then integrated them into a 5 × 5 pixel arrays of sensing matrix fabricated by shadow mask lithography ( Fig. 7b,c ). Each sensing pixel element was extended to two additional contact pads and connected by copper wires. When an irregular object such as a key (6.6 g) was positioned on the top of our sensors, the output current intensity depended on specific locations ( Fig. 7e ). The colour contrast mapped local pressure distribution in consistency with the shape of the key ( Fig. 7f ). 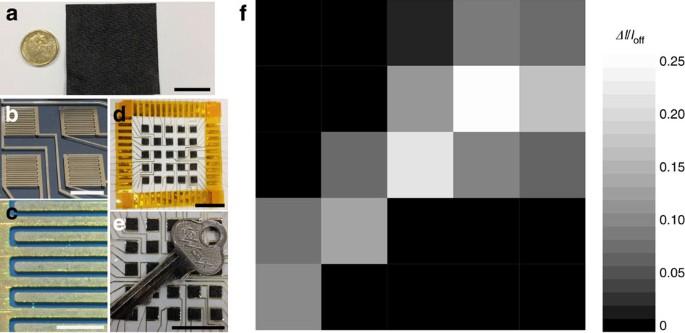Figure 7: Large-area integration and patterning. (a) Photograph of a 5 × 5 cm2gold nanowires-impregnated tissue paper (scale bar, 2 cm). (b) Photograph of interdigitated Ti-Au electrode arrays on PDMS substrate (scale bar, 5 mm). (c) Optical microscope image of one pixel electrode (scale bar, 1 mm). (d) Photograph of a large-area pressure sensor with 5 × 5 pixels (scale bar, 2 cm). (e) Top view of a key (6.6 g) lays on the surface of the 5 × 5 pixel-pressure sensor (scale bar, 2 cm). (f) Current mapping of pressure distributions for the key in (e). Figure 7: Large-area integration and patterning. ( a ) Photograph of a 5 × 5 cm 2 gold nanowires-impregnated tissue paper (scale bar, 2 cm). ( b ) Photograph of interdigitated Ti-Au electrode arrays on PDMS substrate (scale bar, 5 mm). ( c ) Optical microscope image of one pixel electrode (scale bar, 1 mm). ( d ) Photograph of a large-area pressure sensor with 5 × 5 pixels (scale bar, 2 cm). ( e ) Top view of a key (6.6 g) lays on the surface of the 5 × 5 pixel-pressure sensor (scale bar, 2 cm). ( f ) Current mapping of pressure distributions for the key in ( e ). Full size image Generality of our fabrication strategy We found our fabrication approach is general, which could be extended to carbon nanotubes and gold nanorods ( Supplementary Fig. 13 ) as well. However, AuNWs showed the best sensitivity, which is perhaps due to high mechanical flexibility in conjunction with high conductivity. These attribute origins from the unique structures of AuNWs, including the ultra-thinness in width (~2 nm) and the high aspect ratio (>10,000). In summary, we have developed a simple yet efficient, low-cost, bottom-up approach to fabricate a wearable and highly sensitive pressure sensor using ultrathin, high-aspect-ratio AuNWs. This new sensor featured a sensitivity of >1.14 kPa −1 , a fast response time of <17 ms, high stability over >50,000 cycles and a low power consumption of <30 μW when operated under a battery voltage of 1.5 V. With this new sensor, we could detect dynamic forces in a wide pressure range (13~50,000 Pa) with the ability of resolving various complex forces including pressing, bending, torsion and acoustic vibrations. These attributes enabled us to monitor in real-time and in-situ the real-world force signals from radial artery blood pulses and acoustic vibrations. Notably, the entire device fabrication process is scalable without the need of complex and expensive equipment. We believe that our methodologies open a new route to low-cost pressure sensors with potential facile integration into future wearable electronics such as flexible touch-on displays, human–machine interfacing devices and prosthetic skins. Synthesis of ultrathin AuNWs Ultrathin gold nanowires were synthesized as described elsewhere [24] , [25] . In detail, 44 mg HAuCl 4 ·3H 2 O was added into 40 ml hexane (40 ml), followed by addition of 1.5 ml Oleylamine (OA). Note that the gold salts were not dissolved until the addition of OA, which acted as a phase-transfer reagents. After completely dissolving the gold salts, 2.1 ml Triisopropylsilane was added into the above solution. The resulting solution was left to stand for 2 days without stirring at room temperature until the colour turned from yellow into dark red, indicating the formation of AuNWs. The residue chemicals were removed by repeated centrifugation and thorough washing by ethanol/hexane (2/1, v/v) and finally concentrated to a 2 ml stock solution in chloroform. For the entire process, OA molecules played a critical role in dissolving gold salts in Hexane, directing nanowire growth as well as stabilizing AuNWs. Sensor fabrication 8 × 8 mm 2 tissue papers were dipped into a chloroform solution of the AuNWs. After evaporating the chloroform, the colour of tissue paper changed from white to dark red. Then the dip-coating and drying process were repeated for about 10 cycles until the electrical resistance of paper sheets reached to ~2.5 MΩ sq −1 . The Ti/Au interdigitated electrodes (Thickness at 3 nm/30 nm) were deposited onto PDMS substrates (30 × 27 mm 2 ) using a designed shadow mask by an electric beam evaporator (Intlvac Nanochrome II, 10 kV). The spacing between the adjacent electrodes was typically 0.1 mm, with the width of interdigitated electrodes at 0.5 mm. Two 10 × 10 mm 2 contact pads were deposited at the two ends of the interdigitated electrodes to establish external contacts. Then, the bottom layer electrode coated PDMS and upper layer blank PDMS supports were treated by thin oxygen plasma (Harrick Plasma Cleaner PDC-001) and permanently sealed outside the AuNWs coated tissue paper to ensure conformal contact of tissue paper and interdigitated electrodes. Large-area fabrication and patterning A 5 × 5 cm 2 tissue paper was first dipped into the AuNWs stock solution and dried for 10 cycles, leading to a uniform black tissue paper ( Fig. 7a ). Then AuNWs-impregnated paper was cut by paper knife into 4 × 5 mm 2 pieces. In the meantime, a patterned Ti/Au interdigitated electrode arrays on PDMS substrates (65 × 65 mm 2 ) was fabricated using shadow mask lithography mentioned earlier in this work ( Fig. 7b,c ). The spacing and width of electrodes were kept at 100 and 200 μm, with each interdigitated electrode pixel at 5 × 5 mm 2 . Finally, each AuNWs-impregnated paper piece was addressed to the specific electrode pixels and sandwiched between the plasma-treated PDMS sheets, leading to large-area, patterned pressure sensors. Device characterization SEM images were characterized using a JEOL JSM-7001F FEG SEM operated at 5 kV beam voltage. TEM images were carried out using a Philips CM20 TEM at a 200 kV accelerating voltage. Optical images were taken by a Nikon SMZ800 microscope with a Nikon Digital Sight DS-Fi1 camera. The sheet resistances of AuNWs coated tissue papers were carried out on a Jandel four point conductivity probe by using a linear arrayed four point head. The strains were measured by an Instron (Micro Tester, 5848, Instron) using a 100 N load cell and strain control mode with a strain rate of 100% per minute. The current differences and the I–V characteristics for the pressure sensor were recorded by the Parstat 2273 electrochemical system (Princeton Applied Research). For the dynamic force measurement, a computer-based user interface and a micro force sensor (ATI Nano17 Force/Torque Sensor, 1/80 N resolution without filtering) and a Maxon Brushless DC motor using a high resolution quadrature encoder (15 μm of linear resolution) were used to apply an external pressure up to 2,600 Pa with frequency up to 5.5 Hz. For the dynamic low pressure measurement, a piezoelectric stepping positioner (SLC-1730) was used by a custom LabView programme and the force data was measured by an electrical balance (Mettler Toledo NewClassic MF, MS105DU). Materials Gold (III) chloride trihydrate (HAuCl 4 ·3H 2 O, ≥99.9%), Triisopropylsilane (99%) and OA were purchased from Sigma Aldrich. Ethanol, Hexane and chloroform were obtained from Merck KGaA. All chemicals were used as received unless otherwise indicated. All glassware used in the following procedures was cleaned in a bath of freshly prepared aqua regia (highly corrosive!) and rinsed thoroughly in H 2 O before use. Tissue papers were brought from Kimberly-Clark Worldwide Incorporation (Kleenex Brand optimum towel, 30.5 × 24 cm 2 ). PDMS substrates were made by the mixing of the prepolymer gel (Sylgard 184 Silicone Elastomer Base) and the cross linker (Sylgard 184 Silicone Elastomer Curing Agent) at the weight ratio of 10:1. The mixture was poured on a 6″ flat-plate petri dish using 0.5 mm-height shims as spacers and cured at 65 °C for 2 h in an oven. After curing, the PDMS sheet with a thickness of 500 μm was cut into 30 × 27 mm 2 strips for further treatment. The stainless shadow masks were purchased from MasterCut Techniques, Australia. Silver paste was from Dupont (Dupont 4929 N, DuPont Corporation, Wilmington, DE, USA). Aqueous CNT solutions (1 mg ml −1 ) with sodium dodecylbenzenesulphonate (SDBS) (1:10 in quality ratio) as a surfactant were prepared according to the Hu et al . [40] Gold nanorods were synthesized in accordance with our previous work [41] ). How to cite this article: Gong, S. et al. A wearable and highly sensitive pressure sensor with ultrathin gold nanowires. Nat. Commun. 5:3132 doi: 10.1038/ncomms4132 (2014).